Specific recognition of the HIV-1 genomic RNA by the Gag precursor During assembly of HIV-1 particles in infected cells, the viral Pr55 Gag protein (or Gag precursor) must select the viral genomic RNA (gRNA) from a variety of cellular and viral spliced RNAs. However, there is no consensus on how Pr55 Gag achieves this selection. Here, by using RNA binding and footprinting assays, we demonstrate that the primary Pr55 Gag binding site on the gRNA consists of the internal loop and the lower part of stem-loop 1 (SL1), the upper part of which initiates gRNA dimerization. A double regulation ensures specific binding of Pr55 Gag to the gRNA despite the fact that SL1 is also present in spliced viral RNAs. The region upstream of SL1, which is present in all HIV-1 RNAs, prevents binding to SL1, but this negative effect is counteracted by sequences downstream of SL4, which are unique to the gRNA. During assembly, the HIV-1 must select its genomic RNA (gRNA) from a variety of RNAs, including cellular RNAs as well as more than 100 partially or fully spliced viral RNAs (vRNAs) (for recent reviews, see refs 1 , 2 , 3 , 4 , 5 ). HIV-1 gRNA and spliced vRNAs compete for a common packaging pathway, while cellular RNAs are usually packaged with low efficiency, through a different mechanism [6] . It is currently unclear whether discrimination between gRNA and spliced RNA is mediated by the initial binding step to Pr55 Gag , or whether other pathways such as the gRNA nuclear export pathway and subcellular localization are involved [7] , [8] . The Pr55 Gag precursor protein plays a central role in the assembly of HIV-1 virions and in the selection of the gRNA. It consists of the matrix (MA), capsid (CA), nucleocapsid (NC), and p6 or ‘late’ domains; the CA and NC domains, and the NC and p6 domains are separated by the linker peptides p2 and p1, respectively ( Fig. 1a ) [1] , [2] , [3] , [4] , [5] . During or shortly after budding, Pr55 Gag is cleaved by the viral protease to produce the structural proteins of the mature virions: MA, CA and NC. The basic amino acids [9] , [10] and the conserved zinc knuckles [11] , [12] , [13] contribute to the RNA-packaging efficiency and specificity. The mature NCp7 binds RNA with a rather high affinity, but with a relatively low specificity (for reviews, see refs 14 , 15 ) and the solution structure of NCp7 in complex with several HIV-1 RNA motifs have been solved by nuclear magnetic resonance (NMR) [16] , [17] . 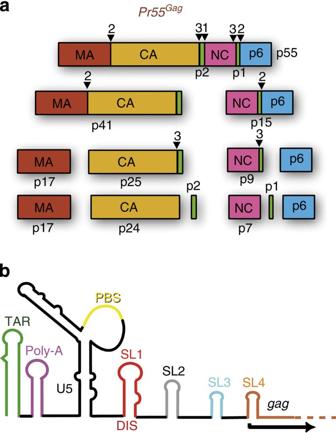Figure 1: Pr55Gagand the 5′-region of HIV-1 gRNA. (a) Functional domains and maturation scheme of HIV-1 Pr55Gag. MA, matrix; CA, capsid; NC, nucleocapsid. (b) Schematic secondary structure model of the 5′-region of the HIV-1 gRNA. TAR,trans-activation response element; Poly-A, stem-loop containing the 5′-copy of the polyadenylation signal in the apical loop; U5, unique in 5′; PBS, primer binding site; DIS, dimerization initiation site; SL1–4: stem-loops 1–4. Figure 1: Pr55 Gag and the 5′-region of HIV-1 gRNA. ( a ) Functional domains and maturation scheme of HIV-1 Pr55 Gag . MA, matrix; CA, capsid; NC, nucleocapsid. ( b ) Schematic secondary structure model of the 5′-region of the HIV-1 gRNA. TAR, trans -activation response element; Poly-A, stem-loop containing the 5′-copy of the polyadenylation signal in the apical loop; U5, unique in 5′; PBS, primer binding site; DIS, dimerization initiation site; SL1–4: stem-loops 1–4. Full size image Interestingly, mouse mammary tumour virus and HIV-1 preferentially package their own gRNA even when the NC domains of these viruses are interchanged [18] , indicating that other Gag domain(s) also contribute to specific packaging of the gRNA. The HIV-1 MA domain binds RNA, and binding of the viral genome may enhance the selectivity of Gag for lipid raft-containing membranes [2] . A mutation in the disordered segment of the carboxy-terminal domain of CA has been shown to reduce RNA packaging [19] . Peptide p2 favours packaging of the gRNA [20] , and mutations in this domain alter packaging of spliced vRNAs [21] , [22] . Finally, deletions or truncations in the p6 domain also reduced the specificity of genomic HIV-1 RNA encapsidation [23] . Pr55 Gag selects HIV-1 gRNA by interacting with packaging signals present on this RNA. An early study [24] showed that the 5′-region of the gRNA, encompassing the R, unique in 5′ (U5), primer binding site (PBS) and leader regions, as well as the first 40 nucleotides of gag are important for packaging. The 5′-region of the HIV-1 gRNA folds into several secondary structure motifs associated with key functions of the retroviral life cycle ( Fig. 1b ) [2] , [3] , [25] . The trans -activation response element (TAR) stem-loop (SL) is essential for Tat-mediated activation of transcription; the poly(A) hairpin contains the 5′-copy of the polyadenylation signal and may also be involved in a long range pseudo-knot [26] ; the PBS domain is crucial for initiation of reverse transcription (RT); SL1 initiates dimerization of the gRNA thanks to the 6-nt self-complementary motif in its loop [2] , [3] , [27] ; SL2 contains the major splice donor site; SL3 is involved in RNA packaging (see below); the unstable SL4 involves the initiation codon of gag and may adopt alternative conformations. The region encompassing SL1 to SL4, usually referred to as ‘Psi’, and especially SL1 and SL3, are required for efficient packaging [6] , [11] , [28] , [29] , [30] , [31] , [32] , [33] . Other studies showed that TAR [34] , the Poly(A) hairpin [35] , [36] and the PBS domain [37] are also required for optimal packaging of the HIV-1 gRNA. Intriguingly, most of the RNA motifs required for efficient packaging are located upstream of SL2 and are thus also present in spliced vRNAs, which are less efficiently packaged into virions ( Fig. 1b ). Long-distance interactions that can only take place in the gRNA [26] , [38] , and especially the so-called U5-AUG interaction, may also contribute to the specificity of gRNA packaging [39] , [40] , while an RNA structural element overlapping the gag-pol frameshift signal may enhance it [41] . The initial recognition of the HIV-1 gRNA by Pr55 Gag , during which discrimination against cellular and spliced vRNAs takes place, occurs in the cytoplasm and involves a very limited number of Pr55 Gag molecules [42] , [43] , [44] , [45] . Once these complexes become anchored in the plasma membrane, Pr55 Gag molecules are rapidly recruited as viral particle assembly proceeds [43] , [46] . Surprisingly, the initial recognition of the gRNA by Pr55 Gag and the mechanism by which this precursor discriminates against spliced vRNAs is still poorly understood. A major hurdle in these studies has been the expression and purification of intact full-length Pr55 Gag . The mature NC domain, truncated forms of the Pr55 Gag precursor, or/and fusion proteins have often been used as a surrogate for Pr55 Gag , as it is very difficult to prevent contamination by proteolysis products. However, whether binding of these proteins to HIV-1 gRNA reflects binding of Pr55 Gag is unknown. Here we study binding of the full-length Pr55 Gag protein to a variety of HIV-1 RNA fragments and mutants. We identify the primary Pr55 Gag binding site on the HIV-1 gRNA and show that Pr55 Gag binding to this site is negatively regulated in spliced vRNAs. Gag expression, purification and characterization Large amounts of Pr55 Gag were produced in Escherichia coli and purified to homogeneity in two high-performance liquid chromatography steps [47] . Suboptimal expression conditions limited incorporation into inclusion bodies and proteolysis, and addition of a C-terminal His 6 -tag allowed efficient separation of the proteolytic cleavage products from the intact protein ( Supplementary Fig. 1a ). Each batch of Pr55 Gag was characterized by dynamic light scattering (DLS). Intensity distribution of Pr55 Gag samples ( Supplementary Fig. 1b ) appeared unimodal and rather monodisperse (polydispersity index=0.22). The mean hydrodynamic radius (Rh=5.8±0.7 nm) was determined via the Stokes–Einstein equation (see Methods), and this was assigned to Pr55 Gag trimers or tetramers. Our DLS data thus indicated that our Pr55 Gag preparations were devoid of microaggregates, which could affect RNA binding studies. Pr55 Gag discriminates between genomic and spliced HIV-1 RNAs We examined whether differential binding to Pr55 Gag could account for the preferential packaging of gRNA versus spliced vRNAs by analysing binding of Pr55 Gag to a series of RNAs corresponding to the first 600 nucleotides of HIV-1 gRNA and spliced RNAs (NL4-3 isolate) using filter-binding assays ( Fig. 2 ). To decrease nonspecific binding of Pr55 Gag to nucleic acids, all experiments were performed in the presence of excess total yeast transfer RNA as competitor, unless stated otherwise. 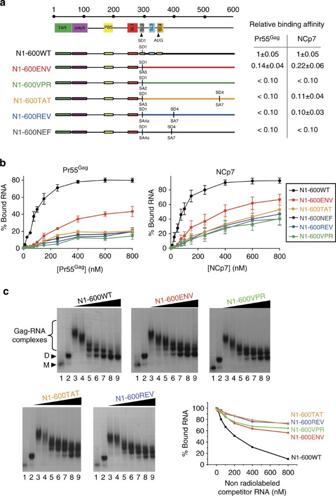Figure 2: Pr55Gagbinding to genomic and spliced HIV-1 RNAs. (a) Schematic drawing of the first 600 nucleotides of genomic and 5 different spliced HIV-1 RNA fragments used. The relative binding affinity of Pr55Gagto these RNAs is indicated on the right. (b) Binding of Pr55Gag(left panel) and mature NCp7 (right panel) to these RNAs was evaluated by filter binding. Data are represented as mean±s.e.m (n=3 or 4). (c) Assessment of the gRNA binding specificity to Pr55Gagusing gel mobility shift assay. Radiolabelled N1-600WT RNA was incubated together with 100 nM Pr55Gagand increasing amounts of unlabelled genomic or spliced vRNA as indicated above the gels. The first two lanes correspond to radiolabelled N1-600WT RNA incubated under denaturing and renaturing conditions, respectively. The concentration of unlabelled competitor RNA in lanes 3 to 9 was 0, 10, 50, 100, 200, 400 and 800 nM, respectively. The last panel presents a quantification of the gels. The fraction of bound RNA corresponds to the sum of all complexes. Figure 2: Pr55 Gag binding to genomic and spliced HIV-1 RNAs. ( a ) Schematic drawing of the first 600 nucleotides of genomic and 5 different spliced HIV-1 RNA fragments used. The relative binding affinity of Pr55 Gag to these RNAs is indicated on the right. ( b ) Binding of Pr55 Gag (left panel) and mature NCp7 (right panel) to these RNAs was evaluated by filter binding. Data are represented as mean±s.e.m ( n =3 or 4). ( c ) Assessment of the gRNA binding specificity to Pr55 Gag using gel mobility shift assay. Radiolabelled N1-600WT RNA was incubated together with 100 nM Pr55 Gag and increasing amounts of unlabelled genomic or spliced vRNA as indicated above the gels. The first two lanes correspond to radiolabelled N1-600WT RNA incubated under denaturing and renaturing conditions, respectively. The concentration of unlabelled competitor RNA in lanes 3 to 9 was 0, 10, 50, 100, 200, 400 and 800 nM, respectively. The last panel presents a quantification of the gels. The fraction of bound RNA corresponds to the sum of all complexes. Full size image The vRNAs bound several Pr55 Gag molecules (see Fig. 2c for the example of N1-600WT, which formed at least four different complexes with Pr55 Gag ), and the actual number of proteins bound to each RNA, as well as their binding mode, might vary between RNAs. In addition, for several RNAs that weakly bound Pr55 Gag , the binding plateau was not reached, even at the maximal Pr55 Gag concentration ( Fig. 2b ). Therefore, we did not attempt to fit the binding curves to theoretical models to derive exact binding parameters. Instead, we determined empirical relative binding affinities of the RNAs compared with a reference (in this case, N1-600WT) by determining the Pr55 Gag concentration required to bind half of the reference RNA bound at the plateau, and dividing it by the Pr55 Gag concentration required to bind the same fraction of each test RNA ( Fig. 2b ). Thus, the relative binding affinities are sensitive to changes in the actual K d and in the binding plateau, which both reflect altered binding compared with the reference RNA. Pr55 Gag bound the gRNA fragment (N1-600WT) efficiently, as half of the plateau was reached at 80±4 nM protein ( Fig. 2b , left panel). By contrast, Pr55 Gag weakly bound singly spliced (N1-600ENV and N1-600VPR) and multiple spliced (N1-600TAT, N1-600REV and N1-600NEF) RNAs ( Fig. 2b , left panel). As the NC domain of Pr55 Gag plays a key role in gRNA packaging, we performed similar experiments with the mature NCp7 protein. Although significant, the discrimination between gRNA and spliced vRNAs by NCp7 was less pronounced ( Fig. 2b , right panel). For instance, at 250 nM protein, Pr55 Gag and NCp7 bound most spliced vRNAs ~10-fold and ~4-fold less efficiently than gRNA, respectively. Interestingly, this difference was due to a decreased binding of Pr55 Gag to the spliced RNAs rather than to increased affinity for gRNA. To obtain more information about the number and relative affinity of the complexes formed between Pr55 Gag and gRNA, we performed competition experiments monitored by band-shift assays ( Fig. 2c ). The gRNA and spliced vRNAs used in this study efficiently dimerized in the binding buffer ( Fig. 2c , lanes 1 and 2 of each gel, which is consistent with previous work [48] ). When radiolabelled N1-600WT RNA was incubated in the presence of 100 nM Pr55 Gag , this RNA was completely shifted ( Fig. 2c , lane 3 of each gel). Concomitant with the addition of unlabelled competitor RNA, the mobility of the N1-600WT RNA/ Pr55 Gag complexes increased and unbound labelled N1-600WT RNA was observed at the highest competitor RNA concentrations. These experiments revealed at least four N1-600WT RNA/Pr55 Gag complexes with different mobilities. In addition, although unlabelled N1-600WT RNA was able to completely displace labelled N1-600WT RNA from the complexes, one (and only one) complex was resistant to displacement by the unlabelled spliced vRNAs ( Fig. 2c , lane 9 of each gel and quantification panel), suggesting that gRNA contains a single high-affinity Pr55 Gag -binding site that is not present in spliced vRNAs. That is, spliced vRNAs can displace weak/nonspecific interactions with Pr55 Gag , but they are unable to displace the high-affinity binding site. Importantly, both gRNA and spliced vRNAs efficiently dimerize via SL1 (ref. 48 ), and Pr55 Gag discrimination between gRNA and spliced vRNAs thus cannot be directly attributed to RNA dimerization. Pr55 Gag binds specifically to SL1 We next analysed binding of Pr55 Gag to the HIV-1 gRNA and its mutants to decipher the molecular basis of the discrimination between gRNA and spliced vRNAs. We first analysed binding of Pr55 Gag to a series of RNA fragments corresponding to different parts of the 5′-region of the gRNA of the NL4-3 HIV-1 isolate using filter-binding assay ( Fig. 3a,b ). 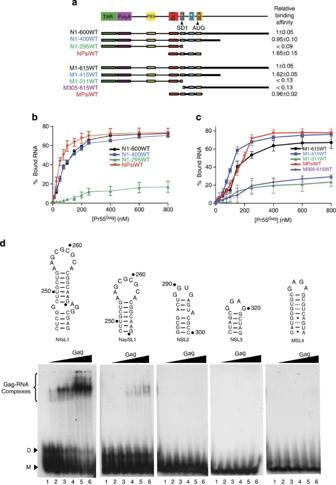Figure 3: Pr55Gagbinding to different regions of the HIV-1 gRNA. (a) Schematic drawing of the gRNA fragments. The binding affinity of Pr55Gagto these RNAs, normalized relative to RNA N1-600WT or M1-615WT, is indicated on the right. Binding of Pr55Gagto large RNAs derived from the gRNA of the NL4-3 (b) and MAL (c) isolates was evaluated by filter binding. Data are represented as mean±s.e.m. (n=3 to 8). (d) Binding of Pr55Gagto the individual SL motifs was analysed by band-shift assays. The structure of the various SL motifs is shown above the gels; two short RNAs corresponding to the apical part of SL1 (NapSL1) and the full-length SL1 (NflSL1) were tested. The Pr55Gagconcentration in lanes 1 to 6 was 0, 50, 100, 200, 400 and 600 nM, respectively. M and D correspond to the monomeric and dimeric species, respectively, of NflSL1 and NapSL1. Figure 3: Pr55 Gag binding to different regions of the HIV-1 gRNA. ( a ) Schematic drawing of the gRNA fragments. The binding affinity of Pr55 Gag to these RNAs, normalized relative to RNA N1-600WT or M1-615WT, is indicated on the right. Binding of Pr55 Gag to large RNAs derived from the gRNA of the NL4-3 ( b ) and MAL ( c ) isolates was evaluated by filter binding. Data are represented as mean±s.e.m. ( n =3 to 8). ( d ) Binding of Pr55 Gag to the individual SL motifs was analysed by band-shift assays. The structure of the various SL motifs is shown above the gels; two short RNAs corresponding to the apical part of SL1 (NapSL1) and the full-length SL1 (NflSL1) were tested. The Pr55 Gag concentration in lanes 1 to 6 was 0, 50, 100, 200, 400 and 600 nM, respectively. M and D correspond to the monomeric and dimeric species, respectively, of NflSL1 and NapSL1. Full size image Pr55 Gag bound with similar affinity to RNAs N1-600WT and N1-400WT, which correspond to the first 600 and 400 nucleotides of the gRNA, respectively. By contrast, Pr55 Gag weakly bound to RNA N1-295WT, which contains all sequences located 5′ to the major splice donor site (in NL4.3, SD1 is located between nucleotides 289 and 290) ( Fig. 3a,b ). Importantly, an RNA corresponding to the region encompassing the SL motifs SL1 to SL4, named NPsiWT, bound Pr55 Gag at least as efficiently as RNAs N1-600WT and N-1-400WT ( Fig. 3a,b ). Next, we performed similar experiments with RNAs derived from the HIV-1 MAL isolate ( Fig. 3a,c ). (For clarity, all RNAs derived from NL4-3 have a name starting with ‘N’, while those derived from MAL have a name starting with ‘M’). The reason for using MAL RNAs is twofold: first, several mutants of this RNA were already available in our laboratory; second, this isolate possesses an insertion 3′ to the PBS that is frequent in the HIV-1 circulating recombinant forms and in subgroup G and A isolates [49] (as a consequence, the SD1 site of the MAL gRNA is located between positions 305 and 306). Importantly, the structural differences in the 5′-region of the gRNA of these two isolates reside in the upper part of the PBS domain [49] . The Psi region of these two gRNAs folds into the same secondary structure motifs (SL1 to SL4). As with the NL4-3 isolate, we observed efficient Pr55 Gag binding to M1-615WT and M1-415WT RNAs, and to an RNA corresponding to the MAL Psi region (MPsiWT), while RNA M1-311WT, corresponding to the sequences upstream of the SD1 site, weakly bound Pr55 Gag . In addition, Pr55 Gag had a weak affinity for RNA M305-615WT, which corresponds to the region downstream of SD1 ( Fig. 3a,c ). Altogether, these experiments demonstrated that the Psi region binds Pr55 Gag specifically and as efficiently as RNA fragments corresponding to at least the first 400 nucleotides of the HIV-1 gRNA. As the Psi region has been proposed to fold into four SLs, we next analysed binding of Pr55 Gag to these individual motifs by band-shift assay. In the absence of competitor, all RNAs, except SL3, bound Pr55 Gag to some degree ( Supplementary Fig. 2 ). However, when excess tRNA was added as competitor, only full-length SL1 bound Pr55 Gag efficiently: Pr55 Gag weakly bound apSL1, while no binding to SL3 and SL4 could be detected ( Fig. 3d ). Thus, SL1 specifically binds Pr55 Gag and the internal loop or/and the lower stem of SL1 are required for efficient binding. The internal loop of SL1 is crucial for Pr55 Gag binding To obtain more precise information about Pr55 Gag binding to the Psi region, we systematically tested by filter-binding assays various SL deletions, apical loop substitutions and internal loop mutations introduced in the context of the NPsi and MPsi RNAs ( Fig. 4a–c ). Each SL was deleted individually, and the last two SLs were also deleted simultaneously ( Fig. 4a ). Substitutions were introduced in the apical loop of each hairpin: a point substitution preventing RNA dimerization [50] was introduced into SL1, a ‘GNRA’ loop was substituted for the SL2 loop and stable ‘UNCG’ loops were substituted for the purine-rich SL3 and SL4 loops ( Fig. 4b ). The internal loop of SL1 was either deleted or replaced by pyrimidines or purines (in NPsiSL1syIL and NPsiSL1srIL, respectively), and the bulge in SL2 was deleted ( Fig. 4c and Supplementary Fig. 3 ). Finally, the lower stem of SL2, which is much more stable than the upper stem, was replaced by a less-stable A–U-rich stem ( Fig. 4c ). 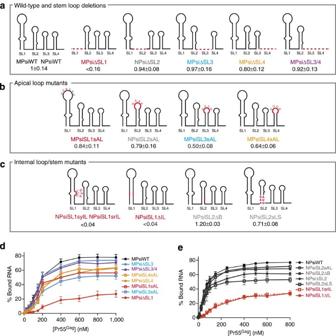Figure 4: Effects of mutations on Pr55Gagbinding to the Psi domain. (a–c) Schematic representation of the mutant RNAs. The mutated regions are indicated in red. The binding affinity of Pr55Gagto these RNAs, normalized relative to RNA MPsiWT or NPsiWT, is indicated under the mutant names. (d,e) Binding curves of Pr55Gagto MAL-derived (d) and NL4-3-derived (e) mutant RNAs. Data are represented as mean±s.e.m. (n=4 to 7). Figure 4: Effects of mutations on Pr55 Gag binding to the Psi domain. ( a – c ) Schematic representation of the mutant RNAs. The mutated regions are indicated in red. The binding affinity of Pr55 Gag to these RNAs, normalized relative to RNA MPsiWT or NPsiWT, is indicated under the mutant names. ( d , e ) Binding curves of Pr55 Gag to MAL-derived ( d ) and NL4-3-derived ( e ) mutant RNAs. Data are represented as mean±s.e.m. ( n =4 to 7). Full size image In line with our previous experiments, deletion of SL1 had a dramatic effect on Pr55 Gag binding, while deletion of the other hairpins had little (≤20%) or no effect ( Fig. 4a,d,e and Supplementary Fig. 3 ). Deleting or substituting the internal loop of SL1 both reduced the relative Pr55 Gag binding affinity more than 25-fold ( Fig. 4c,e and Supplementary Fig. 3 ), while a point substitution in the apical loop that prevents RNA dimerization had a marginal effect ( Fig. 4b,d and Supplementary Fig. 3 ). Deletion of the bulge and destabilization of the lower stem of SL2 had modest but opposite effects, suggesting that a stable SL2 hairpin might slightly favour Pr55 Gag binding ( Fig. 4c,e ). Finally, substitution of the SL3 or SL4 apical loop moderately affected Pr55 Gag binding ( Fig. 4b,d ). Although these experiments clearly point towards the SL1 internal loop as the main determinant of Pr55 Gag binding to the Psi region of both NL4-3 ( Fig. 4 ) and MAL isolates ( Supplementary Fig. 3 ), several studies also indicated that the regions upstream and downstream of the Psi region play a role in RNA packaging [24] , [34] , [35] , [37] , [51] . In addition, tertiary interactions present in the gRNA might be absent in the isolated Psi region [26] , [39] , [40] . Therefore, we introduced the mutations described above in the context of RNAs M1-615 and N1-600, and tested their effect on Pr55 Gag binding using filter-binding assays ( Fig. 5 ). Two different deletions were introduced in SL1: a complete deletion of the hairpin (N1-600ΔflSL1) and a deletion of the upper part of the hairpin that transforms the SL1 internal loop into an apical loop (M1-615ΔapSL1) ( Fig. 5a ). The two substitutions that were introduced in the SL1 apical loop are also different ( Fig. 5a ), but they both impair gRNA dimerization [33] , [50] . Finally, a complete deletion of SL3 was introduced in the RNAs derived from both the MAL and the NL4-3 isolates ( Fig. 5a ). 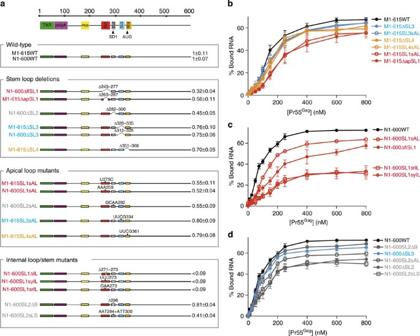Figure 5: Effects of mutations on Pr55Gagbinding to the 5′-region of the HIV-1 genomic RNA (nucleotides 1-600). (a) Schematic representation of the mutant RNAs. The binding affinity of Pr55Gagto these RNAs, normalized relative to RNA M1-615WT or N1-600WT, is indicated on the right. Binding curves of Pr55Gagto MAL-derived (b) and NL4-3-derived (c,d) mutant RNAs. Data are represented as mean±s.e.m. (n=3 to 8). Figure 5: Effects of mutations on Pr55 Gag binding to the 5′-region of the HIV-1 genomic RNA (nucleotides 1-600). ( a ) Schematic representation of the mutant RNAs. The binding affinity of Pr55 Gag to these RNAs, normalized relative to RNA M1-615WT or N1-600WT, is indicated on the right. Binding curves of Pr55 Gag to MAL-derived ( b ) and NL4-3-derived ( c , d ) mutant RNAs. Data are represented as mean±s.e.m. ( n =3 to 8). Full size image Globally, we found that the longer RNAs had similar binding affinities compared with the short RNAs. Even though small context effects exist, mutations in the apical loop of SL2, SL3 and SL4, and mutations in the lower part of SL2, all had limited effects, both in the context of the Psi RNAs and the long RNAs ( Figs 4 and 5 ). When comparing SL deletion mutants, the complete deletion of SL1 had the strongest impact on Pr55 Gag binding. Deletion of the apical part of SL1 resulted in a twofold loss of relative binding affinity, similar to substitutions in the apical loop of SL1 that prevent RNA dimerization ( Fig. 5a–c ), indicating that the upper stem of SL1 is likely to be not directly involved in Pr55 Gag binding, apart from RNA dimerization. Remarkably, substituting pyrimidines or purines for the AGG stretch constituting the 3′-strand of the SL1 internal loop, or deleting this loop dramatically, impaired Pr55 Gag binding ( Fig. 5a,c ). Indeed, these mutations had a significantly more pronounced effect than complete deletion of SL1, raising the possibility that the SL1 internal loop might not directly bind Pr55 Gag but might be involved in a tertiary interaction that is required to expose the primary Pr55 Gag -binding site. However, deletion of SL1 had a more deleterious effect on Pr55 Gag binding than deletion of any other SL, indicating that the lower part of SL1 indeed constitutes a high-affinity Pr55 Gag -binding site. To ensure that loss of Pr55 Gag binding was not due to misfolding of RNA, we compared the structure of N1-600 WT RNA with N1-600ΔflSL1 and N1-600SL1srIL by selective 2′-hydroxyl acylation analysed by primer extension (SHAPE) ( Supplementary Fig. 4 and Supplementary Data 1 ). Our analysis clearly showed that global folding was maintained in mutant RNAs compared with N1-600WT, indicating that our targeted mutagenesis did not lead to misfolding in these mutants ( Supplementary Fig. 4 a,c,d and Supplementary Data 1 ). Furthermore, deletion of SL1 or substitution of the SL1 apical loop impaired RNA dimerization ( Supplementary Fig. 5 ) as expected from previous studies (for review, see ref. 3 ), whereas deletion or substitution of the SL1 internal loop did not inhibit this process ( Supplementary Fig. 5 ), indicating that loss of Pr55 Gag binding was unrelated to effects on RNA dimerization. Visualization of the primary Pr55 Gag binding site The competition experiments described in Fig. 2 revealed that there is a single high-affinity binding site in the HIV-1 gRNA from which Pr55 Gag cannot be readily displaced by spliced vRNAs. To identify this site, we performed footprinting experiments on N1-600WT RNA in the presence of an eightfold molar excess of N1-600VPR RNA using three different chemical probes: benzoyl cyanide (BzCN), which acylates the 2′-hydroxyl of the ribose moiety of any nucleotide in structurally flexible regions; dimethyl sulphate (DMS), which methylates the base of unpaired (or unprotected) A and C residues; and kethoxal, which modifies the base of unpaired G residues. In addition, we used RNase V1, which preferentially cleaves paired or stacked residues and hence is the only probe that gives a positive signal for base-paired residues. In the absence of Pr55 Gag , most RNase V1 cleavages were observed in regions of predicted SL structures, or immediately adjacent to a helix ( Supplementary Fig. 6 ). On addition of increasing concentrations of Pr55 Gag , strong or complete protection against V1 cleavage was noticed 5′ of positions A239, A269, A276, G283, C312, U313, U323 and G331, whereas attenuation of the signal was observed 5′ of G246, G270, G275, G298, C299, A314 and A324 ( Fig. 6a and Supplementary Fig. 6 ). On the other hand, we did not observe any Pr55 Gag -induced RNase V1 cleavage, suggesting that Pr55 Gag binding did not induce formation of new helices in the HIV-1 gRNA. Treatment with BzCN in the absence of Pr55 Gag confirmed the existence of the well-established secondary structure elements present in the 5′-region of the HIV-1 gRNA ( Supplementary Fig. 7 ). Addition of Pr55 Gag induced strong protection of residues G240, G241, G247, G272-G273 and G298, and an attenuation of the SHAPE signal at G285 ( Fig. 6b and Supplementary Fig. 8 ). Unexpectedly, we observed strong Pr55 Gag -induced enhancement of BzCN reactivity at residues A304–A305, U307–U309, G318–A319, A326 and A332, and moderate increase at residues A303, A306, G317 and G329–G331, suggesting that Pr55 Gag destabilized SL3 and the flanking regions ( Fig. 6b and Supplementary Fig. 8 ). Pr55 Gag strongly protected the HIV-1 gRNA against kethoxal modifications at positions G240–G241, G247, G272–G273, G298, G318 and G320, while weaker protections were detected at positions G277–G280, G282–G283, G285 and G317 ( Fig. 6c and Supplementary Fig. 7a ). In addition, footprinting experiments performed with DMS showed protections at residues A242, A276, A293 and A311 ( Fig. 6d and Supplementary Fig. 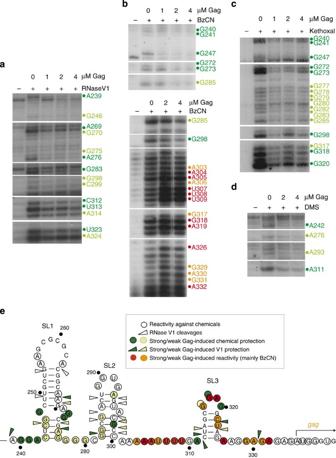Figure 6: Pr55Gagfootprint on HIV-1 genomic RNA. RNA N1-600WT was modified with RNase V1 (a), BzCN (b), kethoxal (c) or DMS (d) in the absence and in the presence of increasing Pr55Gagconcentrations as indicated above each panel. Only portions of the gels in which Pr55Gag-induced reactivity changes were observed are presented; complete gels are presented inSupplementary Figs 6–8. Pr55Gag-induced reactivity changes are summarized ine. 8b ) Figure 6: Pr55 Gag footprint on HIV-1 genomic RNA. RNA N1-600WT was modified with RNase V1 ( a ), BzCN ( b ), kethoxal ( c ) or DMS ( d ) in the absence and in the presence of increasing Pr55 Gag concentrations as indicated above each panel. Only portions of the gels in which Pr55 Gag -induced reactivity changes were observed are presented; complete gels are presented in Supplementary Figs 6–8 . Pr55 Gag -induced reactivity changes are summarized in e . Full size image Altogether, our footprinting experiments indicate that the high-affinity Pr55 Gag binding site consists of the internal loop and the lower stem of SL1 ( Fig. 6e ), in agreement with our filter-binding experiments. It extends to the short single-stranded stretches flanking SL1 and to the lower part of SL2. The latter observation is consistent with the effect of mutations reducing the stability of the lower part of SL2 on Pr55 Gag binding ( Fig. 4 ). In addition, Pr55 Gag induces a destabilization or/and structural rearrangement of SL3 and the single-stranded flanking regions. At the same time, the SL3 loop becomes protected against modifications by kethoxal, suggesting that Pr55 Gag contacts the bases but not the ribose moieties of this loop. Noteworthy, destabilization of a 14-mer SL3 was recently reported on binding of GagΔp6, but not mature NC (ref. 52 ). However, our binding experiments indicate that this contact is not essential for Pr55 Gag binding. Binding of Pr55 Gag to SL1 is regulated by 5′ and 3′ sequences As SL1 is present in all HIV-1 RNA species, a mechanism must exist to limit Pr55 Gag binding to spliced HIV-1 RNAs ( Fig. 2 ). We have observed that Pr55 Gag weakly binds to RNAs N1-295WT and M1-311WT, despite the fact that these RNAs are folded similarly to longer RNAs N1-600WT ( Supplementary Fig. 4a,b ) and M1-707WT (ref. 53 ), and are both capable of dimerization in vitro ( Supplementary Fig. 5 ). This suggests that the sequences located upstream of SL1 inhibit binding of Pr55 Gag to SL1 ( Fig. 3 ). To further investigate this result, we analysed Pr55 Gag binding to RNA fragments starting at position +1 of the gRNA and ending at the end of SL2, SL3 or SL4 ( Fig. 7 ). Surprisingly, none of these RNAs efficiently bound Pr55 Gag ( Fig. 7a ). This was especially unexpected for the RNA fragment N1-SL4WT, as it includes the complete Psi region. An inhibitory effect of the TAR, poly-A and/or PBS domain(s) on Pr55 Gag binding can be clearly observed by comparing Pr55 Gag binding with N1-SL4WT and NPsiWT ( Fig. 7a,b ). Furthermore, the RNA region located between nucleotides 355 (that is, the end of SL4) and 400 suppresses this inhibitory effect, as Pr55 Gag binding was restored in the RNA fragment N1-400WT ( Fig. 7a,b ). To confirm this, we compared Pr55 Gag binding to an RNA fragment starting at SL1 and ending at nucleotide 600 (NSL1-600WT RNA) with N1-600WT RNA ( Fig. 7c ). We found that Pr55 Gag bound the two RNAs with the same efficiency. A similar result was obtained for the MAL isolate ( Supplementary Fig. 9 ). These data show that the Gag open reading frame is not an intrinsic enhancer of Pr55 Gag binding, but indeed acts as a suppressor of the negative upstream element, as we propose in our model ( Fig. 7b ). Importantly, the region between nucleotides 355–400 is only present in gRNA, explaining why HIV specifically selects gRNA even though the high-affinity binding site is present in spliced RNA ( Fig. 7a,b ). 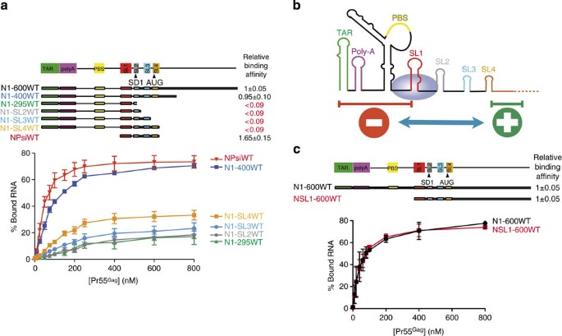Figure 7: Pr55Gagbinding to SL1 is regulated by upstream and downstream sequences. (a) Schematic drawing of the gRNA fragments and relative binding affinity of Pr55Gagto these RNAs normalized to RNA N1-600WT. Binding of Pr55Gagto the NL4-3 gRNA fragments was evaluated by filter binding. Data are represented as mean±s.e.m. (n=3 to 7). (b) Schematic representation of Pr55Gagbinding to HIV-1 gRNA. Pr55Gagbinding to the lower part of SL1 is inhibited by the upstream sequences. This negative regulation is counteracted by a short sequence located 3′ of SL4. (c) Schematic drawing of the gRNA fragments and relative binding affinity of Pr55Gagto N1-600WT and NSL1-600WT RNAs. Binding of Pr55Gagto the NL4-3 gRNA fragments was evaluated by filter binding. Data are represented as mean±s.e.m. (n=3). Figure 7: Pr55 Gag binding to SL1 is regulated by upstream and downstream sequences. ( a ) Schematic drawing of the gRNA fragments and relative binding affinity of Pr55 Gag to these RNAs normalized to RNA N1-600WT. Binding of Pr55 Gag to the NL4-3 gRNA fragments was evaluated by filter binding. Data are represented as mean±s.e.m. ( n =3 to 7). ( b ) Schematic representation of Pr55 Gag binding to HIV-1 gRNA. Pr55 Gag binding to the lower part of SL1 is inhibited by the upstream sequences. This negative regulation is counteracted by a short sequence located 3′ of SL4. ( c ) Schematic drawing of the gRNA fragments and relative binding affinity of Pr55 Gag to N1-600WT and NSL1-600WT RNAs. Binding of Pr55 Gag to the NL4-3 gRNA fragments was evaluated by filter binding. Data are represented as mean±s.e.m. ( n =3). Full size image The SL1 internal loop is a rare motif To evaluate whether the SL1 internal loop could be sufficient to allow discrimination between HIV-1 gRNA and cellular RNAs by Pr55 Gag , we searched for other examples of G/AGG loops in bona fide RNA structures available from public databases. Using the Python framework ‘PyRNA’ ( https://github.com/fjossinet/PyRNA ), 686 X-ray and 77 NMR RNA structures were automatically recovered from the Protein DataBank [54] and annotated with the algorithm RNAVIEW [55] . We performed a similar search for the 2,208 curated seed alignments (44,635 secondary structures) made available with the release of Rfam 11.0 (ref. 56 ). In both cases, apart from the NMR structures of the HIV-1 SL1/DIS and from the Rfam family RF00175 (HIV-1 SL1/DIS), no other RNA structure exhibits such inner loop. These results suggest that the SL1 internal loop may be sufficiently unique to allow Pr55 Gag to discriminate between cellular and vRNAs. Despite a large number a studies, there is no consensus on how Pr55 Gag selects HIV-1 gRNA for packaging. Of note, most previous studies used mature NCp7, intermediate maturation products, truncated forms of Pr55 Gag or/and fusion proteins as a surrogate for Pr55 Gag , and how well these proteins mimic Pr55 Gag is largely unknown. Our data reveal that Pr55 Gag efficiently discriminates between gRNA and spliced HIV-1 RNAs ( Fig. 2 ). The >10-fold reduced binding of Pr55 Gag to spliced RNAs compares well with quantitative packaging studies showing that gRNA is incorporated 50–100-fold more efficiently than spliced RNAs into HIV-1 viral particles [6] . Thus, selection during the initial binding event appears to be the main factor governing selective packaging of the gRNA, even though other pathways such as the gRNA nuclear export pathway and subcellular localization might also play a significant role [7] , [8] . Our RNA binding data is also consistent with the many viral replication studies showing that although the NC domain is crucial for the selectivity of the packaging process, other domains of Pr55 Gag are also involved [18] , [19] , [20] , [21] , [22] , [23] . Our competition experiments revealed the presence of a single high-affinity binding site in the HIV-1 gRNA that is absent from the spliced vRNAs ( Fig. 2 ), in line with recent studies indicating that the initial gRNA selection event involves a very limited number of Pr55 Gag molecules [43] , [44] . Considering the limited impact of substitutions in the SL1 apical loop, which prevent RNA dimerization, on Pr55 Gag binding, there is most likely to be one high-affinity protein-binding site on each RNA molecule constituting the gRNA dimer. These findings allowed us to map this high-affinity Pr55 Gag -binding site by footprinting in the presence competitor spliced vRNA ( Fig. 6 ). Our data showed protections of the internal loop of SL1 and the adjacent regions, in contrast with previous studies that detected much more extended protections, probably corresponding to the sum of specific and nonspecific binding of Gag to the 5′-region of HIV-1 gRNA [57] . Of note, the SL1 internal loop and nucleotides 240–242 immediately 5′ to SL1 were also observed to be strongly protected by the NCp7 zinc knuckles inside viral particles [58] . In line with our footprinting data, our RNA binding data clearly point to the lower part of SL1, and in particular its internal loop, as the primary high-affinity Pr55 Gag -binding site. SL1 is the only SL motif of the Psi region that binds Pr55 Gag with high affinity ( Fig. 3c ), and its internal loop is crucial for Pr55 Gag binding in the context of both Psi and 1-600/1-615 RNAs ( Figs 4 and 5 ). These findings are a priori surprising, as SL1 is present both on gRNA and spliced vRNAs. Indeed, early studies suggested that SL3 was the main packaging signal [11] , [32] , an idea that is still prevalent in the literature. However, these seminal studies were performed before the secondary structure of the Psi region was determined. Consequently, the deletions of SL3 included flanking regions and, in our opinion, it is likely to be that many of the RNA mutants used in these studies adopted aberrant structures. More recent works using exact deletions of SL3 show more modest effects on packaging [6] , [31] , in agreement with our results. Furthermore, our data are totally consistent with the observation that deletions of SL1 have profound effect on gRNA packaging, while substitutions of the SL1 apical loop that affect gRNA dimerization have modest effects [30] , [33] . Interestingly, deletion or substitution of the SL1 internal loop impaired gRNA packaging and reduced viral replication as efficiently as complete deletion of SL1 (ref. 30 ). Of note, the SL1 internal loop is asymmetrical and consists of three guanine and one adenine residues ( Fig. 3d ). NMR structures of NCp7 bound to SL3 and SL2 have demonstrated the key role of guanine residues in the specific binding of the zinc knuckles to RNA [16] , [17] . Similar interactions might confer specificity of Pr55 Gag for the SL1 internal loop. The importance of the lower stem of SL1 for viral replication has also been evaluated in a previous study [59] . Interestingly, out of nine mutants with different complementary sequences that could theoretically form a lower stem, only two displayed no significant replication defect in that study [59] . These results suggest that not only the structure, but also the sequence of the lower SL1 stem might be important for viral replication, although the authors could not exclude that some of the mutant RNAs adopted aberrant conformations [59] . We observed a footprint on this stem on Pr55 Gag binding ( Fig. 6 ), and it is thus conceivable that Pr55 Gag makes sequence-specific contacts with this helix, especially at the junction with the internal loop. We also provided evidence for the existence of a double regulation that ensures selective binding of Pr55 Gag to gRNA, even though SL1 is present in both spliced and gRNA: a negative regulatory element is present in the region encompassing TAR, the poly(A) hairpin, and the PBS domain and a positive regulatory element is defined by nucleotides 355–400 ( Fig. 7 ). As the sequence and structure of the upper part of the PBS domain significantly differ between the HIV-1 NL4.3 and MAL isolates [49] , it is possible that either this region of the RNA is not involved in negative regulation or these two isolates use different mechanisms to negatively regulate Pr55 Gag binding. We suggest that the negative effect is due to steric hindrance that prevents binding of Pr55 Gag to the lower part of SL1 ( Fig. 7 ): this would explain why NCp7 binds more efficiently to the spliced vRNAs than the bulkier Pr55 Gag ( Fig. 2 ). In keeping with the idea that the lower part of SL1 is not accessible to Pr55 Gag in spliced vRNAs, co-transfection of wild type (WT) and SL1-deleted HIV-1 strongly affected packaging of SL1-deleted gRNA, but WT and SL1-deleted spliced vRNAs were packaged with the same efficiency [6] . Although this negative regulation prevents efficient Pr55 Gag binding to spliced vRNAs, selection of the gRNA is ensured by a positive regulation mediated by the region encompassing nucleotides 355–400, which is unique to the gRNA and counteracts the negative impact of the TAR, poly(A) and/or PBS domains. The most probable explanation is that a long-distance interaction between the regions 5′ to SL1 and 3′ to SL4 exposes the lower part SL1 for Pr55 Gag binding. The so-called U5–AUG long-distance interaction was recently proposed to act as a structural switch regulating RNA packaging [40] . The sequences involved in the U5–AUG interaction are all present in RNA N1-SL4WT that weakly bound Pr55 Gag ( Fig. 7 ), and substitution of the SL4 apical loop, which destroys the U5–AUG interaction, had little effect on Pr55 Gag binding ( Figs 4 and 5 ), indicating that the U5–AUG interaction does not regulate the initial Pr55 Gag binding to the gRNA. We suggest that the U5–AUG riboswitch controls later stages of viral particle assembly, as numerous NCp7 proteins are still able to bind the 5′-region of HIV-1 RNA when this interaction is disrupted [40] . Thus, the putative long-range interaction exposing the lower part of SL1 for Pr55 Gag binding remains to be identified. A striking feature emerging from the many gRNA packaging studies is that mutations in each of the structural domains upstream of the gag initiation codon have been reported to affect packaging (TAR [34] , the poly(A) hairpin [35] , [36] , the PBS domain [37] , SL1 (refs 6 , 28 , 30 , 31 , 33 ), SL2 (ref. 31 ) and SL3 (refs 6 , 29 , 30 , 31 )). Reduced gRNA packaging was almost invariably compensated by increased incorporation of spliced vRNA. These observations are consistent with the double regulation of Pr55 Gag binding to SL1 that confer selectivity for the gRNA ( Fig. 7c ). On the one hand, deletion or disruption of TAR, the poly(A) hairpin, or/and the PBS domain might destroy the negative regulatory element that prevents Pr55 Gag binding to spliced vRNAs. On the other hand, mutations either upstream or downstream of SL1 (refs 6 , 29 , 30 , 31 ) that affect the overall three-dimensional structure of the gRNA probably disrupt the putative positive long-distance interaction that optimally exposes the lower part of SL1 for Pr55 Gag binding. If either the positive or the negative regulation is lost, Pr55 Gag would bind gRNA and spliced vRNAs with similar affinity. Pr55 Gag expression, purification and characterization Expression, purification and characterization of NL4.3 Pr55 Gag and GagΔp6 with an appended C-terminal His 6 -tag were performed as recently described [47] . The purity and identity of all protein preparations was confirmed using SDS–PAGE ( Supplementary Fig. 1b ). In addition, Pr55 Gag samples were characterized by DLS in 50 mM Tris–HCl pH 8, 1 M NaCl. The absorbance of the sample was measured and Pr55 Gag concentration was adjusted to 10 μM. Intensities of scattered light and correlation times were measured with a Zetasizer Nano S (Malvern, UK). Measurements were performed in a single 50-μl trUView cuvette (Biorad Laboratories, CA, USA), maintained at 20 °C. Fluctuations of the DLS intensity due to Brownian motion were recorded at microsecond time intervals. An autocorrelation function was derived, thus leading to the determination of diffusion coefficients. Assimilating proteins in solution to spheres, diffusion coefficients were related to the hydrodynamic radius of the particles, R h via the Stokes–Einstein equation: in which k is the Boltzmann constant, T the temperature (°K), μ the solvent viscosity and D is the translational diffusion coefficient. All experimental data were corrected for solvent viscosity (measured with a 3.5-ml micro-Ubbelohde capillary viscosimeter tube from Schott, Germany) and refractive index (measured with an Abbé refractometer). In these buffer conditions the solvent viscosity was 1.1040, cP and the refractive index 1.341. Cloning, mutagenesis, in vitro transcription and RNA purification Several plasmids used for in vitro transcription of WT and mutant RNAs have been described previously [33] , [48] , [50] , [60] ( Supplementary Table 1 ). Additional plasmids were obtained either by PCR cloning or by site-directed mutagenesis using the QuickChange II site-directed mutagenesis kit (Agilent Technologies) ( Supplementary Table 2 ). In vitro transcription and purification of unlabelled RNAs by size-exclusion chromatography was performed as described in refs 33 , 48 , 50 , 60 . Synthetic RNAs corresponding to individual SL motifs were purchased from Microsynth (Switzerland) and purified by HPLC using an anion exchange column (Dionex PA-100). They were labelled using T4 polynucleotide kinase (New England Biolabs) and [γ- 32 P]-ATP (Amersham Biosciences). Internal labelling of longer RNAs was performed by in vitro transcription in the presence of [α- 32 P]-ATP, and purified on a 6% denaturing PAGE gel, as previously described [50] . All labelled RNAs were purified by polyacrylamide gel electrophoresis. RNA-binding assays In a typical filter binding assay, internally labelled HIV-1 RNA (30,000 cpm;<3 nM) and excess total yeast tRNA (2 μg) in 5 μl of Milli-Q water (Millipore) was heated for 2 min at 90 °C and chilled on ice for 2 min with subsequent re-naturation in binding buffer (30 mM Tris–HCl (pH 7.5), 300 mM NaCl, 5 mM MgCl 2 ) supplemented with 5 U of RNasin (Promega) in a final volume of 10 μl for 15 min at 37 °C. In parallel, Pr55 Gag (0–800 nM final concentration) was renatured for 15 min at 22 °C in the binding buffer supplemented with 0.02% (w/v) BSA and 10 mM dithiothreitol, and then added to RNA in a final volume of 60 μl in the presence of 0.01% Triton X-100. After incubation for 30 min at room temperature and 30 min at 4 °C, RNA–protein complexes were loaded onto 0.45 μM pore size cellulose filters (MultiscreenTM 96-well plate, Millipore) pre-soaked with 100 μl of binding buffer and suction filtered through the membrane. Extensive membrane washing (three times with 100 μl of ice-cold binding buffer) was performed to reduce nonspecific binding. Finally, the filters were air-dried and the radioactivity remaining on the filters was determined by liquid scintillation counting using a microplate scintillation counter (Chameleon-Hidex). Alternatively, the membranes were punched out of the filtration plate using Multiscreen Multiple Punch Kit (Millipore) and distributed into scintillation vials for liquid scintillation counting in a Beckman LS 6500 Scintillation Counter. For electrophoretic mobility shift assays, labelled HIV-1 RNA (50,000 cpm;<3 nM) and total yeast tRNA (2 μg) were renatured in binding buffer and incubated with increasing concentrations of Pr55 Gag (0–800 nM) in the presence of 0.01% Triton X-100, 10 mM DTE and 0.02% BSA. After incubation for 30 min at 37 °C and for 30 min at 4 °C, 5 μl of glycerol loading buffer was added, and the reaction mixture was loaded onto native 1% agarose gel. Electrophoresis was performed in TBM (Tris-Borate 0.5 × , MgCl 2 0.1 mM) buffer at 150 V for 5 h at 4 °C with subsequent fixation in 10% trichloroacetic acid for 10 min, drying under vacuum at room temperature and autoradiography. For competition experiments, increasing concentrations of unlabelled competitor RNAs (up to 800 nM) were used and binding was performed with a constant concentration of Pr55 Gag (100 nM) and 50,000 cpm;<3 nM of labelled RNA. Quantitative analysis of the bands corresponding to protein/RNA complexes was performed using ImageGauge software after scanning of the dry gel on a FLA 5000 (Fuji). RNA dimerization assay RNA (200 nM) were prepared in 8 μl of Milli-Q (Millipore). Samples were denatured for 2 min at 90 °C and snap-cooled for 2 min on ice. Dimerization was initiated by addition of 5 × Pr55 Gag binding buffer (final concentration: 30 mM Tris–HCl (pH 7.5), 300 mM NaCl, 5 mM MgCl 2 ) and the samples were incubated for 30 min at 37 °C. Samples were loaded on a 0.8% agarose gel containing ethidium bromide in TBM buffer (0.5 × Tris-Borate, 0.1 mM MgCl 2 ) and run at 150 V for 3 h. For monomer controls, 200 nM RNA was heat denatured for 2 min at 90 °C just before loading. Bands were imaged on a Gel Doc EZ system (BioRad). Probing and footprinting experiments Probing and footprinting experiments were performed on 100 nM N1-600WT RNA in the presence of an eightfold molar excess of N1-600VPR RNA and 2 μg total yeast tRNA. After denaturation and renaturation in the probing buffer in a 20-μl reaction volume, increasing concentrations of Pr55 Gag (0–6 μM) were added and the complexes were incubated for 30 min at 22 °C. DMS modification was performed in 50 mM sodium cacodylate pH 7.5, 300 mM KCl, 5 mM MgCl 2 for 2 or 4 min with 0.8 μl DMS (Fluka) freshly diluted in ethanol (1/20 vol/vol). Kethoxal modification was performed in 50 mM Tris–HCl pH 7.5, 300 mM potassium acetate, 5 mM magnesium acetate with 5–10 μl of kethoxal (United States Biochemicals) freshly dissolved in 20% ethanol (20 mg ml −1 ) for 10 min at room temperature followed by addition of 20 μl 50 mM potassium borate pH 7.0 and 3 μl sodium acetate 3 M. BzCN modification was performed in Hepes-KOH pH 8.0, 300 mM KCl, 5 mM MgCl 2 , with a stock solution of 100 mM BzCN (Sigma-Aldrich) in anhydrous dimethyl sulphoxide (DMSO) added at a 1-μM final concentration and incubated for 1 s at room temperature. Enzymatic digestion with RNase V1 (Ambion) was performed following the manufacturer’s procedure. The RNase V1 concentration was optimized to guarantee one or no statistical cleavage per RNA molecule. Control reactions were performed in the absence of Pr55 Gag and/or the chemical/enzymatic modification reagent. SHAPE methodology The purified in vitro transcribed N1-600WT, N1-295WT, N1-600ΔflSL1 and N1-600SL1srIL RNAs were subjected to h-SHAPE using BzCN. Briefly, 1 pmol of RNA in 8 μl Milli-Q water (Millipore) was denatured for 2 min at 90 °C and then chilled for 2 min on ice. RNA was refolded by the addition of 2 μl 5 × dimer buffer (250 mM sodium cacodylate at pH 7.5; 1.5 M NaCl; 25 mM MgCl 2 ) followed by incubation for 20 min at 37 °C. Next, 2 μg of total yeast tRNA (Sigma-Aldrich) was added to each sample and the volume was adjusted to 15 μl by adding 1 × dimer buffer, and incubated for 10 min at room temperature. Three microlitres of a 1 μM BzCN solution in anhydrous DMSO was used to modify the RNA samples for 1 min, and the reaction was stopped by adding 82 μl water. The negative control samples were treated in the same manner but using only DMSO in the absence of BzCN. All samples were then precipitated using 1 μl of 1 μg μl −1 glycogen solution, 1/10 volume 3 M sodium acetate (pH 6.5) and 3 volumes ethanol for 30 min on dry ice, and the precipitates were collected by centrifugation at 13,000 g for 20 min at 4 °C. The RNA pellets were washed twice with 500 μl cold 80% ethanol to remove salts, dried in a vacuum dryer and dissolved in 7 μl Milli-Q water. Next, to identify the BzCN modification sites, RT was performed on the samples. Two sets of primers were used pAS 267-287: 5′-d (GTC GCC GCC CCT CGC CTC TTG-3′) and pAS 436-457: 5′-d (AGC TCC CTG CTT GCC CAT ACT-3′). These primer sets were labelled with either 6-FAM, VIC, NED or PET. BzCN-modified RNAs were annealed to 1 μl of 1 μM VIC-labelled primer for 2 min at 90 °C and 2 min on ice. After addition of 2 μl 5 × RT buffer (Life Science), the samples were then incubated for 10 min at room temperature. Elongation reaction was performed for 30 min at 42 °C and for 15 min at 50 °C in elongation buffer (1 μl 5 × RT buffer, 3 μl 2.5 mM dNTPs mix, 2 U AMV RT (Life Science) in a total volume of 10.5 μl). For the unmodified RNA samples, 6-FAM-labelled primer were used, and RT reaction was performed in the same manner as for the modified RNA samples. A ddA sequencing ladder was prepared using 2 pmol of untreated RNA and 1 μl of 2 μM NED-labelled primer in 8 μl Milli-Q water. Annealing was performed by heating for 2 min at 90 °C and cooling for 2 min on ice. Two microlitres 10 × RT buffer was added followed by incubation for 15 min at room temperature. The RNA sample was aliquoted into two tubes, and the elongation reaction was performed with 1 μl 10 × RT buffer, 3 μl A10 (0.25 mM dATP, 1 mM dGTP, 1 mM dCTP, 1 mM dTTP), 1 μl of 100 μM ddA and 1 U AMV RT. A ddG ladder was also prepared in the same manner by using PET-labelled primer, G10 (0.25 mM dGTP, 1 mM dATP, 1 mM dCTP, 1 mM dTTP) and 100 μM ddG. All the reactions were stopped by adjusting the volume to 45 μl with water, and proteins were extracted with 50 μl phenol–chloroform. For each experiment, the modified and unmodified samples were pooled with the corresponding ddA and ddG sequencing ladders in a single tube containing 20 μl 3 M sodium acetate and 600 μl ethanol for complementary DNA precipitation. The samples were incubated on dry ice for 30 min, centrifuged at 13,000 g for 20 min at 4 °C, and washed twice with 1 ml cold 80% ethanol. Pellets were dried and resuspended in 10 μl HiDi formamide (ABI), heat denatured at 90 °C and iced for 5 min and centrifuged at 13,000 g for 15 min at 4 °C each before loading on the 96-well plates for sequencing on an Applied Biosystems 3130xl genetic analyser. The results were generated in the form of electropherograms, which were analysed with the SHAPEfinder programme by following the steps prescribed by Vasa et al . [61] RNA structures were drawn using VARNA version 3.9 (ref. 62 ). How to cite this article: Abd El-Wahab, E. W. et al . Specific recognition of the HIV-1 genomic RNA by the Gag precursor. Nat. Commun. 5:4304 doi: 10.1038/ncomms5304 (2014).